Wnt pathway activation by ADP-ribosylation Wnt/β-catenin signalling directs fundamental processes during metazoan development and can be aberrantly activated in cancer. Wnt stimulation induces the recruitment of the scaffold protein Axin from an inhibitory destruction complex to a stimulatory signalosome. Here we analyse the early effects of Wnt on Axin and find that the ADP-ribose polymerase Tankyrase (Tnks)—known to target Axin for proteolysis—regulates Axin’s rapid transition following Wnt stimulation. We demonstrate that the pool of ADP-ribosylated Axin, which is degraded under basal conditions, increases immediately following Wnt stimulation in both Drosophila and human cells. ADP-ribosylation of Axin enhances its interaction with the Wnt co-receptor LRP6, an essential step in signalosome assembly. We suggest that in addition to controlling Axin levels, Tnks-dependent ADP-ribosylation promotes the reprogramming of Axin following Wnt stimulation; and propose that Tnks inhibition blocks Wnt signalling not only by increasing destruction complex activity, but also by impeding signalosome assembly. The Wnt/β-catenin signal transduction pathway directs fundamental processes during metazoan development and tissue homeostasis, whereas deregulation of Wnt signalling underlies numerous congenital disorders and carcinomas [1] , [2] . Two multimeric protein complexes with opposing functions—the cytoplasmic destruction complex and the plasma membrane-associated signalosome—control the stability of the transcriptional co-factor β-catenin to coordinate the state of Wnt pathway activation. In the absence of Wnt stimulation, β-catenin is targeted for proteasomal degradation by the destruction complex, which includes the two tumour suppressors: Axin and Adenomatous polyposis coli (APC), and two kinases: casein kinase 1α (CK1α) and glycogen synthase kinase 3 (GSK3) [3] , [4] , [5] , [6] . Engagement of Wnt with its transmembrane receptors, Frizzled and low-density lipoprotein receptor-related protein 5/6 (herein LRP6), induces rapid LRP6 phosphorylation, recruitment of Axin to phospho-LRP6, and assembly of the signalosome, which includes two other Axin-associated components, GSK3 and Dishevelled (Dvl) [7] , [8] , [9] , [10] , [11] , [12] , [13] , [14] . Signalosome assembly results in the inhibition of β-catenin proteolysis; consequently stabilized β-catenin promotes the transcriptional regulation of Wnt pathway target genes. As a key component in both the destruction complex and the signalosome, Axin is tightly regulated. Under basal conditions, Axin is maintained at very low levels, and serves as the concentration-limiting scaffold for assembly of the destruction complex [15] , [16] . Following Wnt exposure, the rapid association of phospho-Axin with phospho-LRP6 (refs 7 , 12 , 14 ) triggers Axin dephosphorylation, inducing a conformational change that inhibits Axin’s interaction with both the destruction and signalosome complexes [14] , [17] , [18] . Axin is subsequently degraded [7] , [18] , [19] , [20] , [21] , [22] , [23] , [24] ; however, Axin proteolysis occurs several hours after Wnt exposure, and thus does not regulate Axin’s essential role during the initial activation of the Wnt pathway. The mechanisms that rapidly reprogram Axin from inhibitory to stimulatory roles following Wnt exposure remain uncertain. In current models, Wnt stimulation induces Axin’s dissociation from the destruction complex, thereby promoting its interaction with the signalosome [1] , [5] , [6] , [13] , [14] , [18] , [22] , [25] , [26] , [27] . As Wnt stimulation induces Axin dephosphorylation [3] , [18] , [24] , decreased phosphorylation was postulated to facilitate the dissociation of Axin from the destruction complex [17] ; however, recent work revealed that the interaction of Axin with LRP6 precedes Axin dephosphorylation, and that dephosphorylation serves to inhibit, rather than enhance this interaction [14] . Furthermore, some findings have challenged prevailing models, providing evidence that Axin’s interaction with the destruction complex is not diminished upon Wnt stimulation [2] , [19] . Thus, whereas the rapid switch in Axin function following Wnt stimulation is essential for the activation of signalling, the underlying mechanisms remain uncertain. During investigation of this critical process, we have discovered an unanticipated role for the ADP-ribose polymerase Tankyrase (Tnks) in the reprogramming of Axin activity following Wnt exposure. As Tnks-mediated ADP-ribosylation is known to target Axin for proteolysis [28] , small molecule Tnks inhibitors have become lead candidates for development in the therapeutic targeting of Wnt-driven cancers [29] , [30] , [31] . Here we identify a novel mechanism through which Tnks regulates Axin: by promoting Axin’s central role in rapid Wnt pathway activation. We find that Wnt stimulation modulates Axin levels biphasically in both Drosophila and human cells. Unexpectedly, Axin is rapidly stabilized following Wnt stimulation, before its ultimate proteolysis hours later. In an evolutionarily conserved process, the ADP-ribosylated pool of Axin is preferentially increased immediately following Wnt exposure. ADP-ribosylation enhances Axin’s association with phospho-LRP6, providing a mechanistic basis for the rapid switch in Axin function following Wnt stimulation. Our results thus indicate that Tnks inhibition not only increases basal Axin levels, but also impedes the Wnt-dependent interaction between Axin and LRP6, suggesting a basis for the potency of Tnks inhibitors in Wnt-driven cancers. Thus, Tnks not only targets Axin for proteolysis independently of Wnt stimulation, but also promotes Axin’s central role in Wnt pathway activation, which may be relevant to the context-dependent activation of Wnt signalling and the treatment of Wnt-driven cancers with Tnks inhibitors. An in vivo assay for Axin regulation following Wg exposure The precise onset of Wingless (Wg) /Wnt expression in fourteen segmental stripes during early Drosophila embryogenesis has provided a powerful in vivo model for the signalling events triggered by Wg ( Supplementary Fig. 1 ) [32] , [33] . However, previous studies reported contradictory conclusions regarding Axin regulation, with the primary response to Wg exposure described as either Axin proteolysis [23] , or Axin recruitment from cytosol to plasma membrane [34] . Due to technical limitations in these studies, the analysis of Axin was restricted to several hours after the onset of Wg exposure. In addition, Axin was overexpressed at levels high enough to abrogate Wg signalling, which disrupts physiological regulation. We reasoned that the conflicting conclusions in previous reports might have resulted from these experimental barriers. Therefore, we sought to develop a system that would permit an in vivo analysis of Axin at near-physiological levels immediately following Wg stimulation. Because endogenous levels of Axin in Drosophila embryos are too low to be visualized with Axin antibodies, we generated transgenes encoding Axin tagged with a V5 epitope ( Axin-V5) , and used site-specific integration [35] , [36] coupled with the UAS/Gal4 system [37] to direct their expression at near-physiological levels. Expression of Axin-V5 during early embryogenesis was induced with a maternal α-tubulin enhancer ( mat-Gal4 ) that drives ubiquitous transcription [38] . In Axin null mutant embryos, Wg signalling is aberrantly activated throughout the ectoderm [39] , as revealed by the ectopic expression of both engrailed and wg ( Supplementary Fig. 2a–h ). Expression of Axin-V5 in Axin null mutants completely prevented this constitutive activation of the Wg pathway, and critically, did not disrupt normal signalling ( Supplementary Fig. 2i–n ). Thus, Axin-V5 replaced the function of endogenous Axin, and was expressed at levels that were regulated physiologically. Further, in wild-type embryos expressing Axin-V5 , the segmentally striped pattern of Wg, the resultant stabilization of Armadillo (Arm)/β-catenin in Wg-responding cells [40] , the Wg-dependent expression of engrailed [41] , [42] , and the specification of Wg-dependent cell fates, as revealed by the patterning of the larval cuticle [43] , were normal ( Supplementary Fig. 3a–h ). To compare the relative levels of Axin-V5 and endogenous Axin, we examined embryonic lysates. Detection of endogenous Axin by immunoblotting of cell extracts had not been possible with existing Axin antibodies [18] . Therefore, we generated a new Axin antibody that allowed sensitive detection of endogenous Axin, and confirmed its specificity using RNAi-mediated Axin knockdown ( Supplementary Fig. 3i ). We used this Axin antibody to immunoblot lysates from wild-type embryos expressing Axin-V5 ( Supplementary Fig. 3j ). Axin-V5 was distinguished from endogenous Axin by its slower migration rate in electrophoresis, resulting from the V5 tag. Immunoblotting revealed that Axin-V5 was not overexpressed relative to the level of endogenous Axin; instead, Axin-V5 levels were lower than the level of endogenous Axin both before and after the onset of Wg expression ( Supplementary Fig. 3j–l ). We conclude that Axin levels were increased by less than twofold following the expression of Axin-V5. Biphasic regulation of Axin following Wg and Wnt exposure Thus, expression of these Axin transgenes in wild-type embryos enabled an in vivo analysis of Axin at near-physiological levels before, during, and after the onset of Wg stimulation. We found that during the first 3 h of embryogenesis, before and during the onset of Wg expression, Axin was distributed uniformly throughout the ectoderm ( Figs 1a–l and 2a–c ). However, within 30 min after the onset of Wg expression in segmental stripes, a major change in Axin was observed, starting in late stage 8 and persisting throughout stage 9. Axin was no longer distributed uniformly, but instead was present in wide segmental stripes of increased intensity ( Fig. 1m–r ; Supplementary Fig. 4 ). The Axin fluorescence intensity in these stripes was two- to threefold higher than that in the interstripes ( Supplementary Fig. 4 ). Moreover, the temporal appearance of the Axin stripes was coincident with the stabilization of Arm/β-catenin in segmental stripes [40] ( Supplementary Figs 5d–f and 6a–c ), suggesting that the Axin stripes were an early indicator of the initial cellular response to Wg stimulation. 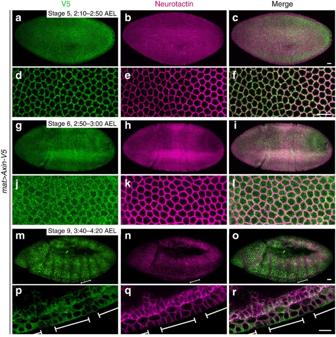Figure 1: Rapid appearance of Axin in segmental stripes following Wg exposure. (a–l) Axin is distributed uniformly in the embryonic ectoderm before and at the onset of Wingless (Wg) expression. Confocal images of embryos expressingAxin-V5driven by themat-Gal4driver. Genotype left, antibodies top. Embryonic stage and developmental time in hours after egg lay (AEL) are indicated at the top right ofa,gandm. Anterior left, dorsal up. In stage 5 and 6 embryos, Axin-V5 and the transmembrane protein Neurotactin are distributed uniformly throughout the ectoderm (a–l). Higher magnification images (d–fandj–l). (m–r) Axin is distributed in segmental stripes after the onset of Wg expression. By stage 9, Axin-V5 accumulates in segmental stripes with increased staining intensity (m–o). Higher magnification images (p–r). White bars indicate the width of a single Axin stripe. Scale bar, 25 μm. Figure 1: Rapid appearance of Axin in segmental stripes following Wg exposure. ( a – l ) Axin is distributed uniformly in the embryonic ectoderm before and at the onset of Wingless (Wg) expression. Confocal images of embryos expressing Axin-V5 driven by the mat-Gal4 driver. Genotype left, antibodies top. Embryonic stage and developmental time in hours after egg lay (AEL) are indicated at the top right of a , g and m . Anterior left, dorsal up. In stage 5 and 6 embryos, Axin-V5 and the transmembrane protein Neurotactin are distributed uniformly throughout the ectoderm ( a – l ). Higher magnification images ( d – f and j – l ). ( m – r ) Axin is distributed in segmental stripes after the onset of Wg expression. By stage 9, Axin-V5 accumulates in segmental stripes with increased staining intensity ( m – o ). Higher magnification images ( p – r ). White bars indicate the width of a single Axin stripe. Scale bar, 25 μm. 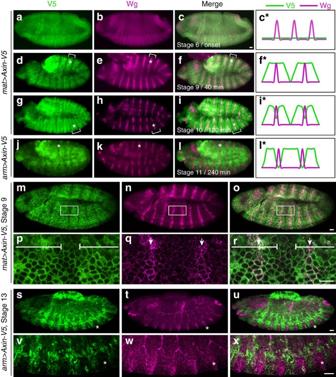Figure 2: Axin is rapidly stabilized and subsequently destabilized following Wg exposure. (a–c) Axin is distributed uniformly in the ectoderm at the onset of Wg exposure. Embryos expressingAxin-V5driven bymat-Gal4 (mat>Axin-V5)stained with V5 and Wg antibodies. Stage of embryonic development and corresponding time relative to the onset of Wg expression is indicated at bottom left ofc,f,i,l. At 3 h of development (stage 6), Axin-V5 is distributed uniformly throughout the embryonic ectoderm and the initial expression of Wg in segmental stripes is weak. (d–f) Axin levels increase rapidly following Wg exposure. By 30 to 40 min after the onset of Wg expression (late stage 8 to stage 9), Axin-V5 is distributed in wide segmental stripes (indicated by brackets) that overlap the narrow Wg stripes (asterisks). (g–l) Axin levels subsequently decrease, beginning at 2 h after Wg exposure. (g–i) Approximately 120 min after onset of Wg expression, mid-stage 10 embryos. During this transitional stage, the Axin-V5 level is decreased precisely at the position of the Wg stripes (asterisks), but remains elevated in the neighbouring cells (brackets). (j–l) Embryos expressingAxin-V5driven byarm-Gal4 (arm>Axin-V5)stained with V5 and Wg antibodies.arm-Gal4drives ubiquitous transcription at late embryonic stages, and thus allows analysis of Axin regulation in stage 11 embryos. By 240 min after the onset of Wg exposure, the Axin-V5 level is markedly decreased at the position of the Wg stripes. Wg (asterisks) and Axin stripes are spatially juxtaposed. (c*–l*) Schematic illustration of the spatial relationship between Axin-V5 and Wg with respect to the onset of Wg exposure. (m–r) Axin levels increase rapidly in response to Wg exposure. Confocal images of stage 9 embryo (m–o) and higher magnification images of boxed region (p–r). Axin stripes (white bars) are centered directly over Wg expressing cells (arrows). (s–x) Axin levels are decreased by several hours after Wg exposure. Confocal images of stage 13 embryo expressingAxin-V5with thearm-Gal4driver. By this time, Axin and Wg stripes are spatially juxtaposed (s–u), as shown in higher magnification images (v–x). Asterisks indicate the position of Wg stripe. For all images, anterior left, dorsal up. Scale bar, 25 μm. Full size image Figure 2: Axin is rapidly stabilized and subsequently destabilized following Wg exposure. ( a – c ) Axin is distributed uniformly in the ectoderm at the onset of Wg exposure. Embryos expressing Axin-V5 driven by mat-Gal4 (mat>Axin-V5) stained with V5 and Wg antibodies. Stage of embryonic development and corresponding time relative to the onset of Wg expression is indicated at bottom left of c , f , i , l . At 3 h of development (stage 6), Axin-V5 is distributed uniformly throughout the embryonic ectoderm and the initial expression of Wg in segmental stripes is weak. ( d – f ) Axin levels increase rapidly following Wg exposure. By 30 to 40 min after the onset of Wg expression (late stage 8 to stage 9), Axin-V5 is distributed in wide segmental stripes (indicated by brackets) that overlap the narrow Wg stripes (asterisks). ( g – l ) Axin levels subsequently decrease, beginning at 2 h after Wg exposure. ( g – i ) Approximately 120 min after onset of Wg expression, mid-stage 10 embryos. During this transitional stage, the Axin-V5 level is decreased precisely at the position of the Wg stripes (asterisks), but remains elevated in the neighbouring cells (brackets). ( j – l ) Embryos expressing Axin-V5 driven by arm-Gal4 (arm>Axin-V5) stained with V5 and Wg antibodies. arm-Gal4 drives ubiquitous transcription at late embryonic stages, and thus allows analysis of Axin regulation in stage 11 embryos. By 240 min after the onset of Wg exposure, the Axin-V5 level is markedly decreased at the position of the Wg stripes. Wg (asterisks) and Axin stripes are spatially juxtaposed. ( c *– l *) Schematic illustration of the spatial relationship between Axin-V5 and Wg with respect to the onset of Wg exposure. ( m – r ) Axin levels increase rapidly in response to Wg exposure. Confocal images of stage 9 embryo ( m – o ) and higher magnification images of boxed region ( p – r ). Axin stripes (white bars) are centered directly over Wg expressing cells (arrows). ( s – x ) Axin levels are decreased by several hours after Wg exposure. Confocal images of stage 13 embryo expressing Axin-V5 with the arm-Gal4 driver. By this time, Axin and Wg stripes are spatially juxtaposed ( s – u ), as shown in higher magnification images ( v – x ). Asterisks indicate the position of Wg stripe. For all images, anterior left, dorsal up. Scale bar, 25 μm. Full size image To determine the relative position of the segmental stripes of Axin and Wg, we co-stained embryos expressing Axin-V5 with V5 and Wg antibodies. Within 30 min after the onset of Wg expression in segmental stripes, all Axin stripes were centered over Wg stripes ( Fig. 2d–f,m–r ; Supplementary Fig. 5a–c ). As Wg is not required for embryonic segmentation [43] , we tested whether Wg was important for generating the segmental stripes of Axin. In contrast with wild-type embryos, no Axin stripes were observed in wg null mutants; instead, the Axin-V5 staining was uniform ( Supplementary Fig. 6d–g ). Thus, Wg is required for the differential regulation of Axin in the embryonic ectoderm. To rule out the possibility that the segmental Axin stripes were caused artifactually by the V5 epitope tag, we generated transgenic flies expressing GFP-tagged Axin; Axin-GFP was also expressed using the mat-Gal4 driver. Before, during, and after the onset of Wg expression, the Axin-GFP and Axin-V5 patterns were identical, as were the kinetics of Wg-dependent changes in their distribution ( Supplementary Fig. 7 ). These data supported the hypothesis that within 30 min after Wg exposure, Axin is tightly regulated in Wg-responding cells, and that the rapid appearance of Axin in stripes of increased intensity coincides with the initial activation of the pathway. To further test this hypothesis, we examined endogenous Axin levels in lysates from wild-type embryos. Embryos were collected at developmental stages that just preceded (1.5 to 2.5 h of development) or followed (3.5 to 4.5 h of development) the onset of Wg expression. To monitor the initial activation of the Wg pathway, we examined the accumulation of phosphorylated Arrow/LRP6 with an antibody directed against phosphothreonine 1572 in human LRP6 (ref. 44 ), a residue that is conserved in Drosophila ( Supplementary Fig. 8a ). RNAi-mediated arrow knockdown in S2R+ cells confirmed the specificity of this signal ( Supplementary Fig. 8b,c ). After the onset of Wg stimulation, phospho-Arrow levels increased and remained elevated ( Supplementary Fig. 9a ). We found that Axin levels increased by approximately threefold after Wg stimulation ( Supplementary Fig. 9a,b ; stage 9). The increase in Axin levels likely resulted from increased protein stability, as the Axin gene is not a transcriptional target of the Wg pathway, and instead Axin transcripts are expressed ubiquitously [39] . These findings provided further evidence that Axin is unexpectedly stabilized following Wg stimulation, and supported the kinetics of Axin stabilization observed in the embryos by immunostaining. In addition, we found that after the initial increase in Axin during the early response to Wg exposure, Axin levels subsequently decreased ( Supplementary Fig. 9a,b ; stage 13, 9h 20 min to 10h 20 min of development), as reported previously for mammalian Axin [18] , [19] , [22] , [23] , [24] . To investigate the kinetics of this process, we examined the in vivo pattern of embryonic Axin stripes. We found that the Axin stripes persisted for 80 to 100 min following Wg exposure ( Fig. 2d–f,m–r ; Supplementary Figs 5a–c and 7m–o ; late stage 8 to stage 9). After that time, Axin levels decreased, initially in cells exposed to the highest levels of Wg ( Fig. 2g–i , 2 h following Wg exposure; mid-stage 10), and subsequently, in their neighbours ( Fig. 2j–l,s–x , 4 h following Wg exposure; Stage 11-13). Thus, when Axin was stabilized in the early phase following Wg exposure, Axin and Wg stripes overlapped ( Fig. 2d–f,m–r ; Supplementary Figs 5a–c and 7m–o ). By contrast, when Axin was destabilized in the delayed phase, Axin and Wg stripes were spatially juxtaposed ( Fig. 2j–l,s–x ), as observed previously [23] . In summary, our unprecedented ability to visualize Axin before, during, and after the onset of Wg exposure revealed that Axin is regulated biphasically in response to Wg stimulation in vivo , which reconciles the contradictory conclusions in previous reports [23] , [34] . To determine whether the biphasic regulation of Axin in response to Wg stimulation is evolutionarily conserved, we examined Axin1 levels in cultured human cells exposed to Wnt ( Supplementary Fig. 9c–f ). Treatment of two cell lines, HEK293T or SW480, with Wnt3A protein resulted in rapid pathway activation, with the accumulation of phospho-LRP6 within 15 to 30 min ( Supplementary Fig. 9c,e ). In both cell lines, the levels of endogenous Axin1 protein increased within 15 to 30 min following Wnt3A treatment ( Supplementary Fig. 9c–f ). This increase in Axin1 likely resulted from increased protein stability, as the Axin1 gene is not a transcriptional target of the Wnt pathway [45] , [46] , and the increased Axin1 protein level was observed within 15 min of Wnt exposure. By 2 h after Wnt treatment, Axin1 levels decreased ( Supplementary Fig. 9c–f ), as reported previously [18] , [24] . These findings suggested that the initial stabilization and subsequent destabilization of Axin in response to Wnt exposure, and the kinetics of this response, are evolutionarily conserved. Tnks promotes Axin stabilization following Wg exposure As Tnks is known to target Axin for proteolysis [28] , we sought to determine whether Tnks regulates Axin before and/or following Wg exposure. The Tnks-dependent proteolysis of Axin requires direct interaction of Tnks with a small region in the Axin amino terminus, the Tnks-binding domain (TBD; refs 28 , 47 , 48 ). To determine whether the evolutionarily conserved TBD facilitates the degradation of Drosophila Axin, we generated an Axin-V5 transgene with a 21 amino-acid deletion that eliminates the TBD (AxinΔTBD; Supplementary Fig. 10a,b ). To enable their direct comparison, the Axin-V5 and AxinΔTBD-V5 transgenes were integrated at the same genomic site ( attP33) , and were expressed using the same mat-Gal4 driver. By comparison with Axin-V5, the levels of AxinΔTBD were increased by three- to fourfold ( Supplementary Fig. 10c–g ), even before the onset of Wg expression (0–2 h of embryogenesis, up to stage 4; Supplementary Fig. 10c–e ). We conclude that the TBD is important to control the basal levels of Drosophila Axin independently of Wg exposure. To determine whether the TBD has additional roles in Axin regulation following Wg exposure, we analysed embryos expressing AxinΔTBD after the onset of Wg expression. Unexpectedly, and in contrast with Axin-V5 ( Fig. 3a–c ), AxinΔTBD-V5 was not present in segmental stripes 30 min after Wg exposure; instead, AxinΔTBD levels were increased uniformly in all ectodermal cells ( Fig. 3g–i ; Supplementary Fig. 11a–c ; late stage 8 and stage 9). Thus, the early stripes of Axin that form in response to Wg exposure were dependent on the TBD; deletion of the TBD resulted in the aberrant Axin stabilization in all cells. 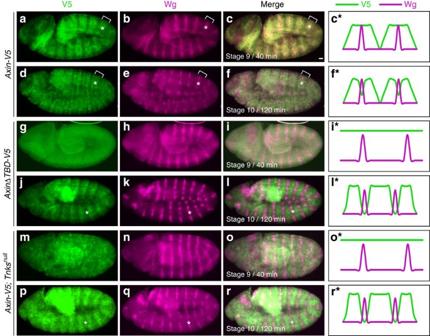Figure 3: Tnks promotes Axin regulation during the early phase, but is dispensable for Axin proteolysis during the delayed phase after Wg exposure. (a-f) Wild-type Axin is initially stabilized and subsequently degraded following Wg exposure. Stage 9 and mid-stage 10 embryos expressingAxin-V5driven by themat-Gal4driver, co-stained with V5 and Wg antibodies. Genotypes left, antibodies top. (a–c) By 40 min after the onset of Wg exposure (stage 9), Axin-V5 is distributed in wide segmental stripes (brackets) that overlap narrow Wg stripes (asterisks). (d–f) By 120 min after the onset of Wg exposure (mid-stage 10), Axin-V5 staining is decreased in cells expressing Wg (asterisks). (g–l) The Tnks-binding domain in Axin is required for the initial stabilization of Axin induced by Wg exposure, but dispensable for the subsequent Wg-dependent Axin proteolysis. (g–i) In stage 9 embryos, AxinΔTBD-V5 staining is uniformly high throughout the embryonic ectoderm; no segmental stripes are present. (j–l) In mid-stage 10 embryos, the AxinΔTBD-V5 levels are decreased in cells expressing Wg (asterisks). Axin stripes are spatially juxtaposed with Wg stripes. (m–r) Tnks is required for the initial stabilization of Axin induced by Wg exposure, but dispensable for the subsequent Wg-dependent Axin proteolysis. (m–o) In stage 9Tnksnull mutant embryos, Axin-V5 staining is uniformly high in all ectodermal cells. (p–r) In mid-stage 10Tnksnull mutant embryos, Axin-V5 is decreased in cells expressing Wg (asterisks). Axin stripes are spatially juxtaposed with Wg stripes. Scale bar, 25 μm. Schematic illustration of spatial relationship of Axin-V5 and Wg with respect to the onset of Wg expression inc*–r*. Figure 3: Tnks promotes Axin regulation during the early phase, but is dispensable for Axin proteolysis during the delayed phase after Wg exposure. ( a - f ) Wild-type Axin is initially stabilized and subsequently degraded following Wg exposure. Stage 9 and mid-stage 10 embryos expressing Axin-V5 driven by the mat-Gal4 driver, co-stained with V5 and Wg antibodies. Genotypes left, antibodies top. ( a – c ) By 40 min after the onset of Wg exposure (stage 9), Axin-V5 is distributed in wide segmental stripes (brackets) that overlap narrow Wg stripes (asterisks). ( d – f ) By 120 min after the onset of Wg exposure (mid-stage 10), Axin-V5 staining is decreased in cells expressing Wg (asterisks). ( g – l ) The Tnks-binding domain in Axin is required for the initial stabilization of Axin induced by Wg exposure, but dispensable for the subsequent Wg-dependent Axin proteolysis. ( g – i ) In stage 9 embryos, AxinΔTBD-V5 staining is uniformly high throughout the embryonic ectoderm; no segmental stripes are present. ( j – l ) In mid-stage 10 embryos, the AxinΔTBD-V5 levels are decreased in cells expressing Wg (asterisks). Axin stripes are spatially juxtaposed with Wg stripes. ( m – r ) Tnks is required for the initial stabilization of Axin induced by Wg exposure, but dispensable for the subsequent Wg-dependent Axin proteolysis. ( m – o ) In stage 9 Tnks null mutant embryos, Axin-V5 staining is uniformly high in all ectodermal cells. ( p – r ) In mid-stage 10 Tnks null mutant embryos, Axin-V5 is decreased in cells expressing Wg (asterisks). Axin stripes are spatially juxtaposed with Wg stripes. Scale bar, 25 μm. Schematic illustration of spatial relationship of Axin-V5 and Wg with respect to the onset of Wg expression in c *– r *. Full size image To determine whether the TBD is also required for the subsequent degradation of Axin induced by Wg, we examined embryos at later developmental stages ( Fig. 3j–l ). By comparison with their neighbours, the levels of AxinΔTBD were decreased in Wg-responding cells 2 h after Wg exposure, with kinetics similar to those observed for wild-type Axin ( Fig. 3d–f,j–l ; Supplementary Fig. 12i–k ; mid-stage 10). These findings indicated that the TBD is not required for the Wg-dependent proteolysis of Axin. Therefore, we hypothesized that Tnks facilitates the stabilization of Axin following Wg exposure, but is dispensable for the subsequent Axin degradation. To test this hypothesis, we examined Tnks null mutant embryos expressing Axin-V5 . In contrast with wild-type embryos, no early stripes of Axin were present in Tnks mutants; instead, Axin levels were uniformly high throughout the embryonic ectoderm ( Fig. 3m–o ; Supplementary Fig. 11d–f ). Two hours after Wg exposure, the levels of Axin decreased in Wg-responding cells in Tnks mutants, as we had observed in wild-type embryos ( Fig. 3d–f,p–r ). Thus, the same phenotype was present in embryos expressing AxinΔTBD or in Tnks null mutant embryos: the early Axin stripes were absent, whereas the late Axin stripes were present. These data indicated that in the absence of Tnks, the initial Wg-dependent regulation of Axin did not occur, and Axin was aberrantly stabilized in all cells, but that the subsequent Wg-dependent Axin proteolysis occurred with normal kinetics. To determine whether the regulation of Axin at the earliest times after Wg exposure promotes activation of the Wg pathway, we analysed the expression of the transcription factor Engrailed. During early embryogenesis, the initial transcription of engrailed is not dependent on Wg; however, Wg signalling is required subsequently to maintain engrailed expression [41] , [42] . The expression of engrailed is among the earliest readouts for the activation of Wg signalling. Upon expression of Axin-V5 in either wild-type or Axin null mutant embryos, both the onset and maintenance of engrailed expression in segmental stripes were normal ( Fig. 4a,b and Supplementary Fig. 2m ; compare with Supplementary Fig. 2b ). In contrast, upon expression of AxinΔTBD-V5 in either wild-type or Axin null mutant embryos, the initiation of engrailed expression was normal, but the maintenance of engrailed expression was markedly diminished, as revealed by the decreased width of Engrailed stripes ( Fig. 4c,d ; Supplementary Fig. 12m ), indicating defects in Wg signalling. Similarly, examination of larval cuticles following expression of Axin-GFP revealed normal epidermal patterning, in which regions of naked cuticle alternated between ventral segmental denticle belts ( Supplementary Fig. 13a ). In contrast, a segment polarity phenotype was observed upon expression of AxinΔTBD-GFP ( Supplementary Fig. 13b ), in which the ventral epidermis formed denticles in place of naked cuticle [43] . These findings suggested that Tnks promotes not only the initial Wg-dependent regulation of Axin, but also the activation of Wg signalling. 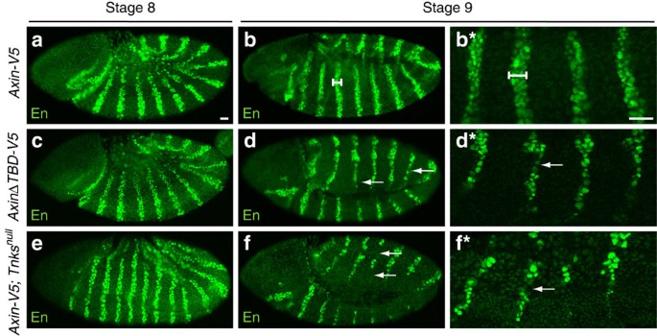Figure 4: Tnks promotes the activation of Wg signalling. Tnks and the TBD in Axin promote Wg signalling. Confocal images of stage 8 or 9 embryos stained with Engrailed (En) antibody. Genotypes left, developmental stage indicated on top. (a,b) In wild-type embryos expressingAxin-V5, En is present in stripes that are 2 to 3 cells in width (b*, white bar), at both 10 min after the onset of Wg expression (stage 8) and 40 min after the onset of Wg (stage 9). (c,d) In embryos expressingAxinΔTBD-V5, the initiation of En stripes (stage 8) is normal (c), but En stripes decay in 68% (n=50) of embryos (d), as revealed by the aberrantly narrowed width by stage 9 (d*, arrow). (e,f) InTnksnull mutant embryos expressingAxin-V5, En expression is normal at stage 8 (e), but decays by stage 9 in 75% (n=36) of embryos (f*, arrow). Images inb*,d* andf* are higher magnification views of embryos inb,d, andfrespectively. In all images, anterior left, dorsal up. Scale bar, 25 μm. Figure 4: Tnks promotes the activation of Wg signalling. Tnks and the TBD in Axin promote Wg signalling. Confocal images of stage 8 or 9 embryos stained with Engrailed (En) antibody. Genotypes left, developmental stage indicated on top. ( a , b ) In wild-type embryos expressing Axin-V5 , En is present in stripes that are 2 to 3 cells in width ( b *, white bar), at both 10 min after the onset of Wg expression (stage 8) and 40 min after the onset of Wg (stage 9). ( c , d ) In embryos expressing AxinΔTBD-V5 , the initiation of En stripes (stage 8) is normal ( c ), but En stripes decay in 68% ( n =50) of embryos ( d ), as revealed by the aberrantly narrowed width by stage 9 ( d *, arrow). ( e , f ) In Tnks null mutant embryos expressing Axin-V5 , En expression is normal at stage 8 ( e ), but decays by stage 9 in 75% ( n =36) of embryos ( f *, arrow). Images in b *, d * and f * are higher magnification views of embryos in b , d , and f respectively. In all images, anterior left, dorsal up. Scale bar, 25 μm. Full size image We tested this hypothesis by examining Wg pathway activation in Tnks null mutant embryos expressing Axin-V5 . In Tnks mutant embryos expressing Axin-V5 , the initiation of engrailed expression was normal ( Fig. 4e ; stage 8), but its maintenance was markedly disrupted ( Fig. 4f ; stage 9). Therefore, the same defects in Wg pathway activation were observed in Tnks mutant embryos expressing Axin-V5 and in wild-type embryos expressing AxinΔTBD-V5 . Nonetheless, no defects in engrailed expression were observed in Tnks mutants ( Supplementary Fig. 14 ), and these mutants were viable under standard laboratory conditions [49] , [50] , [51] . These findings revealed that a less than twofold increase in Axin levels by the expression of Axin-V5 ( Supplementary Fig. 3l ) uncovers the importance of Tnks in promoting Wg signalling during embryogenesis, and suggested that the regulation of Axin by Tnks following Wg exposure can be functionally compensated until Axin reaches a critical threshold level. Altogether, these findings indicated that Tnks promotes not only the stabilization of Axin after Wg exposure, but also the activation of Wg signalling. Tnks promotes Wg signalling through a novel mechanism We sought to elucidate the mechanism through which Tnks regulates Axin and the activation of Wg signalling. In the current model, Tnks promotes Axin degradation, limiting the activity of the destruction complex, and thereby facilitating the activation of Wg signalling [28] . Alternatively, Tnks might also regulate the rapid transition of Axin following Wg stimulation. To distinguish between these two possibilities, we tested whether an increase in the basal levels of Axin, comparable to the higher levels present in AxinΔTBD or in Tnks mutants, was sufficient to inhibit Axin regulation or Wg pathway activation. We generated transgenic flies in which the Axin-V5 transgene was integrated at a different site in the genome ( attP40 ), which is known to result in higher expression levels than the original site ( attP33 ) [35] . Indeed, immunoblotting of lysates revealed that the basal levels of Axin in embryos expressing Axin-V5 integrated at the attP40 site were significantly higher than the Axin levels in embryos expressing either Axin-V5 or AxinΔTBD integrated at the attP33 site ( Fig. 5a,b ). Similarly, comparison of fluorescence intensity revealed that levels of attP40 Axin-V5 were higher than attP33 Axin-V5, attP33 AxinΔTBD-V5 , or Tnks null mutant embryos expressing attP33 Axin-V5 ( Supplementary Fig. 15 ). 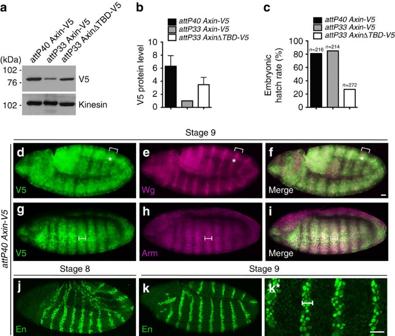Figure 5: In addition to its known role in Axin proteolysis, Tnks promotes Wg pathway activation through a novel mechanism of Axin regulation. (a-b) Generation of transgenic flies with wild-type Axin at levels higher than those resulting from loss of Tnks-dependent Axin proteolysis. (a) Immunoblot analysis of lysates from embryos expressing eitherAxin-V5orAxinΔTBD-V5integrated at theattP33or theattP40site. Lysates were prepared from embryos collected at 0–2 h of development, before the onset of Wg expression. Levels of V5 fromattP33 AxinΔTBD-V5are higher thanattP33 Axin-V5when expressed under the same conditions. Integration of the wild-typeAxin-V5transgene at a different genomic site,attP40, results in levels that are higher thanattP33 AxinΔTBD-V5. Kinesin was used as a loading control. (b) Quantification of relative levels of indicated protein from experiments shown ina. Error bars represent s.e.m. of three independent experiments.P=0.0348 (one-way ANOVA with Kruskal–Wallis test). (c) The hatch rate of embryos expressingattP40 Axin-V5,attP33 Axin-V5orattP33 AxinΔTBD-V5with themat-Gal4driver. By comparison with embryos expressingattP33 Axin-V5orattP40 Axin-V5, the hatch rate is reduced by expression ofattp33 AxinΔTBD-V5. At least 200 embryos of each genotype were analysed, as indicated. (d–i) An increase in wild-type Axin, above the levels resulting from loss of Tnks-dependent Axin proteolysis, is compatible with the rapid stabilization of Axin following Wg exposure. (d–f) In stage 9 embryos expressingattP40 Axin-V5driven bymat-Gal4, Axin-V5 accumulates in segmental stripes (brackets) that overlap the Wg stripes (asterisks). (g–i) Co-staining with V5 and Arm antibodies shows that Axin-V5 accumulates normally in Wg-responding cells, as revealed by co-localization with cells that accumulate Arm (white bars). (j,k) An increase in wild-type Axin, above the levels resulting from loss of Tnks-dependent Axin proteolysis, is compatible with the activation of Wg signalling. En expression is normal at both stage 8 (j) and stage 9 (k). A higher magnification view of the En stripes inkis shown (k*, white bar indicates the width of a single En stripe). Scale bar, 25 μm. Figure 5: In addition to its known role in Axin proteolysis, Tnks promotes Wg pathway activation through a novel mechanism of Axin regulation. ( a - b ) Generation of transgenic flies with wild-type Axin at levels higher than those resulting from loss of Tnks-dependent Axin proteolysis. ( a ) Immunoblot analysis of lysates from embryos expressing either Axin-V5 or AxinΔTBD-V5 integrated at the attP33 or the attP40 site. Lysates were prepared from embryos collected at 0–2 h of development, before the onset of Wg expression. Levels of V5 from attP33 AxinΔTBD-V5 are higher than attP33 Axin-V5 when expressed under the same conditions. Integration of the wild-type Axin-V5 transgene at a different genomic site, attP40 , results in levels that are higher than attP33 AxinΔTBD-V5 . Kinesin was used as a loading control. ( b ) Quantification of relative levels of indicated protein from experiments shown in a . Error bars represent s.e.m. of three independent experiments. P =0.0348 (one-way ANOVA with Kruskal–Wallis test). ( c ) The hatch rate of embryos expressing attP40 Axin-V5 , attP33 Axin-V5 or attP33 AxinΔTBD-V5 with the mat-Gal4 driver. By comparison with embryos expressing attP33 Axin-V5 or attP40 Axin-V5 , the hatch rate is reduced by expression of attp33 AxinΔTBD-V5 . At least 200 embryos of each genotype were analysed, as indicated. ( d – i ) An increase in wild-type Axin, above the levels resulting from loss of Tnks-dependent Axin proteolysis, is compatible with the rapid stabilization of Axin following Wg exposure. ( d – f ) In stage 9 embryos expressing attP40 Axin-V5 driven by mat-Gal4 , Axin-V5 accumulates in segmental stripes (brackets) that overlap the Wg stripes (asterisks). ( g – i ) Co-staining with V5 and Arm antibodies shows that Axin-V5 accumulates normally in Wg-responding cells, as revealed by co-localization with cells that accumulate Arm (white bars). ( j , k ) An increase in wild-type Axin, above the levels resulting from loss of Tnks-dependent Axin proteolysis, is compatible with the activation of Wg signalling. En expression is normal at both stage 8 ( j ) and stage 9 ( k ). A higher magnification view of the En stripes in k is shown ( k *, white bar indicates the width of a single En stripe). Scale bar, 25 μm. Full size image However, despite the increased levels of Axin present in embryos expressing attP40 Axin-V5 , the early regulation of Axin in Wg-responding cells, as revealed by the position, width and timing of appearance of the Axin stripes, was the same in embryos expressing either attP40 Axin-V5 or attP33 Axin-V5 ( Fig. 5d-i , compare with Fig. 2d–f and Supplementary Fig. 6a–c ). Further, both the initiation and the maintenance of engrailed expression were similar in embryos expressing either attP33 Axin-V5 or attP40 Axin-V5 , as was the embryonic hatch rate ( Fig. 5c,j,k , compare with Fig. 4a,b ). These results were in sharp contrast with the absence of early Axin stripes, the disrupted engrailed expression, and the decreased embryonic hatch rate in embryos expressing AxinΔTBD or in Tnks mutants expressing attP33 Axin-V5 ( Figs 3g–i,m–o and 4c–f ; Supplementary Fig. 12l–n ; Fig. 5c ). Altogether, these findings demonstrate that the level to which Axin is increased in Tnks mutant embryos expressing Axin-V5 is not sufficient to disrupt Axin regulation or to inhibit Wg signalling. Instead, these results suggested that in addition to its known role in Axin proteolysis, Tnks also acts through a distinct mechanism to promote the initial regulation of Axin and the activation of signalling following Wg exposure. Wnt stimulation increases the ADP-ribosylated Axin level Our unanticipated findings suggested that Tnks-mediated ADP-ribosylation of Axin facilitates rapid Axin regulation and the activation of signalling following Wnt exposure. To test this hypothesis, we examined whether Wnt stimulation modulates the levels of ADP-ribosylated Axin. Detection of ADP-ribosylated Axin has been challenging, as the levels are very low under basal conditions [52] , and ADP-ribosylation does not markedly alter the electrophoretic mobility of Axin [28] , [52] . Therefore, to detect ADP-ribosylated Axin, we utilized a previously developed pull down assay based on the Trp–Trp–Glu (WWE) domain of the RING-type E3 ubiquitin ligase RNF146/Iduna coupled to glutathione S -transferase (GST) [52] . Tnks and RNF146 are known to form a stable complex that targets substrates for ADP-ribosylation and subsequent ADP-ribose-dependent ubiquitination [52] , [53] , [54] , [55] . The WWE domain of RNF146 interacts directly with the poly(ADP-ribose) in these Tnks substrates to promote their ubiquitination. As a control for specificity of the GST-WWE assay, pull downs were simultaneously performed using a GST-WWE R164A mutant control, in which an arginine to alanine substitution in the RNF146 WWE domain abolishes interaction with poly(ADP-ribose) [52] . As an additional control for specificity, we generated a construct that encodes mouse Axin1 with a nine amino-acid deletion in the TBD, Axin1ΔTBD , which is predicted to prevent the Tnks-dependent ADP-ribosylation of Axin1 (refs 28 , 47 , 48 ). GST-WWE pull downs were performed with lysates from HEK293T cells expressing either Flag-Axin1 or Flag-Axin1ΔTBD , followed by immunoblotting with Flag antibody ( Fig. 6a ). Although the levels of Axin1 and Axin1ΔTBD in these lysates were comparable, GST-WWE pulled down Axin1, but not Axin1ΔTBD. Further, neither Axin1 nor Axin1ΔTBD was pulled down by the GST-WWE R164A control. Tnks-mediated ADP-ribosylation does not markedly alter the electrophoretic mobility of Axin [28] , [52] ; nonetheless, we detected small mobility shifts in the ADP-ribosylated Axin isolated by GST-WWE pull down ( Supplementary Fig. 16a ), suggesting that Axin is pulled down through its ADP-ribosylation, rather than through association with another ADP-ribosylated protein. These findings confirmed the specificity of the GST-WWE pull-down assay for the detection of ADP-ribosylated Axin. 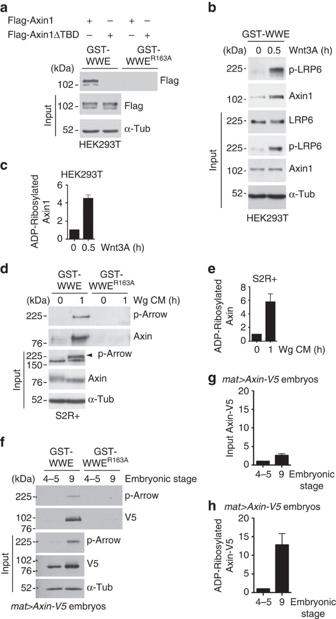Figure 6: ADP-ribosylated Axin rapidly accumulates following Wnt stimulation. (a) Use of a GST-WWE pull down assay for specific detection of ADP-ribosylated Axin. Detection of ADP-ribosylated mouse Flag-Axin1 and Flag-Axin1ΔTBD using either GST-WWE or GST-WWER163Acontrol pull downs in HEK293T cells. Flag-Axin1 is pulled down by GST-WWE; however, the Flag-Axin1ΔTBD control is not. (b,c) The levels of ADP-ribosylated Axin rapidly increased following Wnt exposure in human cells. (b) HEK293T cells were treated with Wnt3A for 0.5 h, and cell lysates were subsequently pulled down by GST-WWE followed by immunoblot analysis with the indicated antibodies. Following treatment with Wnt, phospho-LRP6 is pulled down by GST-WWE. (c) Quantification of relative ADP-ribosylated Axin1 levels from experiments shown in (b). Error bars represent s.e.m. of three independent experiments.P=0.0062 (Student’st-test). (d,e) The level of ADP-ribosylated Axin rapidly increased following Wg exposure inDrosophilacells. (d) Immunoblot of lysates from S2R+ cells treated with Wg conditioned medium (CM) for 1 h and then subjected to GST-WWE pull down. Treatment with Wg CM increased the level of ADP-ribosylated Axin pulled down with GST-WWE. Following treatment with Wg CM, phospho-Arrow is pulled down by GST-WWE. (d, input) Treatment with Wg CM induced a mobility shift in Axin. (e) Quantification of relative levels of ADP-ribosylated Axin from experiments shown in (d). Error bars represent s.e.m. of four independent experiments.P=0.0147 (Student’st-test). (f–h) The levels of Axin-V5 and ADP-ribosylated Axin-V5 are rapidly increased after the onset of Wg stimulation inDrosophilaembryos. Embryos at stages 4–5 and stage 9 expressingAxin-V5driven by themat-Gal4driver. Stages 4-5 (1.5 to 2.5 h of development) are before the onset of Wg stimulation and stage 9 (3.5 to 4.5 h of development) is after the onset of Wg stimulation. Lysates were immunoblotted by indicated antibodies, followed by GST-WWE pull down. Axin-V5 and phospho-Arrow are pulled down by GST-WWE following Wg stimulation. (gandh) Quantification of relative Axin-V5 and ADP-ribosylated Axin-V5 levels from experiments shown in (f). (g)P=0.0321 (Student’st-test). (h)P=0.0305 (Student’st-test). Error bars represent s.e.m. of three independent experiments. Figure 6: ADP-ribosylated Axin rapidly accumulates following Wnt stimulation. ( a ) Use of a GST-WWE pull down assay for specific detection of ADP-ribosylated Axin. Detection of ADP-ribosylated mouse Flag-Axin1 and Flag-Axin1ΔTBD using either GST-WWE or GST-WWE R163A control pull downs in HEK293T cells. Flag-Axin1 is pulled down by GST-WWE; however, the Flag-Axin1ΔTBD control is not. ( b , c ) The levels of ADP-ribosylated Axin rapidly increased following Wnt exposure in human cells. ( b ) HEK293T cells were treated with Wnt3A for 0.5 h, and cell lysates were subsequently pulled down by GST-WWE followed by immunoblot analysis with the indicated antibodies. Following treatment with Wnt, phospho-LRP6 is pulled down by GST-WWE. ( c ) Quantification of relative ADP-ribosylated Axin1 levels from experiments shown in ( b ). Error bars represent s.e.m. of three independent experiments. P =0.0062 (Student’s t -test). ( d , e ) The level of ADP-ribosylated Axin rapidly increased following Wg exposure in Drosophila cells. ( d ) Immunoblot of lysates from S2R+ cells treated with Wg conditioned medium (CM) for 1 h and then subjected to GST-WWE pull down. Treatment with Wg CM increased the level of ADP-ribosylated Axin pulled down with GST-WWE. Following treatment with Wg CM, phospho-Arrow is pulled down by GST-WWE. ( d , input) Treatment with Wg CM induced a mobility shift in Axin. ( e ) Quantification of relative levels of ADP-ribosylated Axin from experiments shown in ( d ). Error bars represent s.e.m. of four independent experiments. P =0.0147 (Student’s t -test). ( f – h ) The levels of Axin-V5 and ADP-ribosylated Axin-V5 are rapidly increased after the onset of Wg stimulation in Drosophila embryos. Embryos at stages 4–5 and stage 9 expressing Axin-V5 driven by the mat-Gal4 driver. Stages 4-5 (1.5 to 2.5 h of development) are before the onset of Wg stimulation and stage 9 (3.5 to 4.5 h of development) is after the onset of Wg stimulation. Lysates were immunoblotted by indicated antibodies, followed by GST-WWE pull down. Axin-V5 and phospho-Arrow are pulled down by GST-WWE following Wg stimulation. ( g and h ) Quantification of relative Axin-V5 and ADP-ribosylated Axin-V5 levels from experiments shown in ( f ). ( g ) P =0.0321 (Student’s t -test). ( h ) P =0.0305 (Student’s t -test). Error bars represent s.e.m. of three independent experiments. Full size image To determine whether Wnt stimulation induces changes in the level of endogenous ADP-ribosylated Axin, we performed GST-WWE pull downs on lysates from HEK293T cells treated with Wnt3A protein. The accumulation of phospho-LRP6 was used to monitor activation of the Wnt pathway ( Fig. 6b , input). Unexpectedly, within 30 min of Wnt3A exposure, the level of ADP-ribosylated Axin1 increased by four- to fivefold ( Fig. 6b,c ). These results demonstrate that the pool of ADP-ribosylated Axin increases rapidly following Wnt exposure. To determine whether the increase in the pool of ADP-ribosylated Axin in response to Wnt exposure is an evolutionarily conserved process, we used GST-WWE pull downs to analyse lysates from Drosophila S2R+ cells treated with Wg conditioned medium ( Fig. 6d ). We analysed two downstream signalling events to monitor the temporal response of these cells to Wg exposure: the phosphorylation of Arrow/LRP6 (refs 8 , 56 ), and the stabilization of Arm/β-catenin [40] , [57] ( Supplementary Fig. 8d ). Treatment of S2R+ cells with Wg conditioned medium resulted in increased levels of phospho-Arrow within 10 min, which peaked at 40 to 50 min and remained elevated for more than 2 h. In addition, Arm/β-catenin was stabilized within 20 min of Wg exposure and remained elevated for 2 h ( Supplementary Fig. 8d ), as reported previously [57] . Our new Axin antibody allowed sensitive detection of endogenous Axin, and revealed a mobility shift following Wg stimulation ( Figs 6d and 7a , input), consistent with the Wnt-dependent dephosphorylation of Axin observed previously in mammalian cells [14] , [17] , [18] . GST-WWE pull down followed by immunoblotting with the Axin antibody revealed that the levels of ADP-ribosylated Axin increased within one hour of stimulation with Wg. In contrast, Axin was not pulled down by the GST-WWE R164A control, confirming specificity of the signal ( Fig. 6d ). The increase in ADP-ribosylated Axin levels ranged from four- to sevenfold, indicating that, as observed in human cells, ADP-ribosylated Axin accumulated rapidly following Wg stimulation in Drosophila cells ( Fig. 6d,e ). 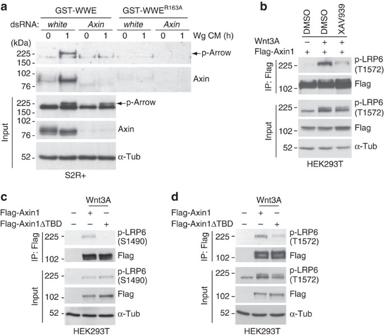Figure 7: ADP-ribosylation enhances interaction of Axin with phospho-LRP6 following Wnt stimulation. (a) Phospho-Arrow interacts with ADP-ribosylated Axin following Wg exposure. Immunoblot of S2R+ cells treated with dsRNA againstAxinorwhite(negative control), then treated with Wg CM for 1 h, subjected to GST-WWE pull down, and analysed by immunoblotting with indicated antibodies. Treatment with Wg CM markedly increases the amount of ADP-ribosylated Axin pulled down with GST-WWE, but not the GST-WWER163Acontrol. On treatment with Wg CM, phospho-Arrow is also pulled down with GST-WWE, but not the GST-WWER163Acontrol. The pull down of phosphorylated Arrow by GST-WWE is prevented by treatment withAxindsRNA. (a, input) Treatment with Wg CM induced a mobility shift in Axin. There is a small decrease in the level of phospho-LRP6 followingAxinknockdown. These data suggest that in Drosophila, Axin is not essential for Wg-dependent phosphorylation of LRP6, but may facilitate this process. (b) ADP-ribosylation enhances the interaction of Axin with phospho-LRP6. HEK293T cells expressingFlag-Axin1were treated with either the DMSO control or the small molecule Tnks inhibitor XAV939 for 24 h. XAV939 diminishes the Wnt3A-dependent interaction between Axin1 and phospho-LRP6. (c,d) The Tnks-binding domain enhances the interaction of Axin with phospho-LRP6 following Wnt exposure. HEK293T cells transfected with either Flag-Axin1 or Flag-Axin1ΔTBD, and subsequently treated with Wnt3A for 30 min. Lysates were immunoprecipitated by Flag antibody, followed by immunoblot using indicated antibodies. Both (c) phospho-LRP6 (S1490) and (d) phospho-LRP6 (T1572) antibodies demonstrate that Axin1 interacts with phospho-LRP6 following Wnt3A stimulation; however, deletion of the TBD of Axin1 diminishes this interaction. α-Tub was used as a loading control. These experiments were performed at least three times with representative results shown. Figure 7: ADP-ribosylation enhances interaction of Axin with phospho-LRP6 following Wnt stimulation. ( a ) Phospho-Arrow interacts with ADP-ribosylated Axin following Wg exposure. Immunoblot of S2R+ cells treated with dsRNA against Axin or white (negative control), then treated with Wg CM for 1 h, subjected to GST-WWE pull down, and analysed by immunoblotting with indicated antibodies. Treatment with Wg CM markedly increases the amount of ADP-ribosylated Axin pulled down with GST-WWE, but not the GST-WWE R163A control. On treatment with Wg CM, phospho-Arrow is also pulled down with GST-WWE, but not the GST-WWE R163A control. The pull down of phosphorylated Arrow by GST-WWE is prevented by treatment with Axin dsRNA. ( a , input) Treatment with Wg CM induced a mobility shift in Axin. There is a small decrease in the level of phospho-LRP6 following Axin knockdown. These data suggest that in Drosophila, Axin is not essential for Wg-dependent phosphorylation of LRP6, but may facilitate this process. ( b ) ADP-ribosylation enhances the interaction of Axin with phospho-LRP6. HEK293T cells expressing Flag-Axin1 were treated with either the DMSO control or the small molecule Tnks inhibitor XAV939 for 24 h. XAV939 diminishes the Wnt3A-dependent interaction between Axin1 and phospho-LRP6. ( c , d ) The Tnks-binding domain enhances the interaction of Axin with phospho-LRP6 following Wnt exposure. HEK293T cells transfected with either Flag-Axin1 or Flag-Axin1ΔTBD, and subsequently treated with Wnt3A for 30 min. Lysates were immunoprecipitated by Flag antibody, followed by immunoblot using indicated antibodies. Both ( c ) phospho-LRP6 (S1490) and ( d ) phospho-LRP6 (T1572) antibodies demonstrate that Axin1 interacts with phospho-LRP6 following Wnt3A stimulation; however, deletion of the TBD of Axin1 diminishes this interaction. α-Tub was used as a loading control. These experiments were performed at least three times with representative results shown. Full size image To further test this hypothesis in vivo , we quantitated changes in the levels of ADP-ribosylated Axin following Wg stimulation in lysates from staged Drosophila embryos expressing Axin-V5 using GST-WWE pull downs. These studies revealed that the total levels of Axin-V5 increased by approximately threefold in stage 9 embryos (after Wg stimulation) by comparison with stage 4–5 embryos (before Wg stimulation; Fig. 6f,g ). Importantly, the level of ADP-ribosylated Axin-V5 increased by ∼ 13-fold after Wg stimulation ( Fig. 6f,h ). As described above, small mobility shifts were detected in ADP-ribosylated Axin ( Supplementary Fig. 16b ). These results indicated that the pool of ADP-ribosylated Axin is preferentially increased following Wg exposure. Therefore, we conclude that the rapid increase in ADP-ribosylated Axin is an evolutionarily conserved response to Wnt/Wg stimulation. ADP-ribosylation enhances the interaction of Axin with LRP6 On the basis of the rapid accumulation of ADP-ribosylated Axin in both Drosophila and human cells following Wnt exposure, we speculated that ADP-ribosylation of Axin might facilitate Axin’s interaction with phospho-LRP6 and the subsequent activation of the Wnt pathway. Indeed, we observed that in lysates of human cells exposed to Wnt, not only Axin, but also phospho-LRP6 was pulled down by GST-WWE ( Fig. 6b ). Analogously, in lysates of Drosophila cultured cells or embryos exposed to Wg, phospho-Arrow was pulled down by GST-WWE, but not the GST-WWE R164A control, indicating a requirement for ADP-ribosylation ( Fig. 6d,f ). Thus, we hypothesized that both phospho-LRP6 and phospho-Arrow were pulled down through their association with ADP-ribosylated Axin following Wnt exposure. To test this hypothesis, we repeated the GST-WWE pull downs after depleting Drosophila Axin using RNAi-mediated knockdown in cultured Drosophila cells ( Fig. 7a ). Treatment of S2R+ cells with Axin dsRNA resulted in a marked reduction in Axin levels, to the extent that Arm/β-catenin was aberrantly stabilized in the absence of Wg stimulation ( Supplementary Fig. 3i ). In the presence or absence of Axin knockdown, the level of phospho-Arrow was comparable ( Fig. 7a , input); however, the pull down of phospho-Arrow by GST-WWE was completely dependent on Axin ( Fig. 7a ). Although we cannot exclude the possibility that phospho-LRP6/Arrow is ADP-ribosylated in an Axin-dependent manner, these findings support the hypothesis that following Wg exposure, phospho-Arrow interacts with ADP-ribosylated Axin. To further test the hypothesis that the ADP-ribosylation of Axin promotes its interaction with phospho-LRP6 following Wnt stimulation, we treated HEK293T cells expressing Flag-Axin1 with either a dimethyl sulfoxide (DMSO) control or with the small molecular inhibitor XAV939 (ref. 28 ), to inhibit the catalytic activity of the two human Tnks proteins. We immunoprecipitated from lysates of these cells with Flag antibody, followed by immunoblotting with phospho-LRP6 antibodies. Treatment with XAV939, but not the DMSO control, markedly decreased the Wnt-dependent interaction between Axin1 and phospho-LRP6 within 30 min of Wnt3A exposure ( Fig. 7b ). To further test this hypothesis, we immunoprecipitated lysates of HEK293T cells expressing Flag-Axin1 or Flag-Axin1ΔTBD with Flag antibody, followed by immunoblotting with phospho-LRP6 antibodies directed against either phospho-serine S1490 [S1490 (ref. 8 )] or phosphothreonine 1572 [T1572 (ref. 44 )]. By 30 min after treatment with Wnt3A, Axin1 interacted with phospho-LRP6, as revealed by both phospho-LRP6 antibodies ( Fig. 7c,d ) [8] , [12] . In contrast, deletion of the TBD in Axin1 diminished the interaction of Axin with phospho-LRP6 ( Fig. 7c,d ). Analogously, deletion of the TBD in Drosophila Axin decreased the Wg-dependent interaction between Axin and phospho-Arrow ( Supplementary Fig. 17a ). Deletion of the TBD in human Axin1 had no detectable effect on Axin1’s interaction with GSK3β, β-catenin or Dvl ( Supplementary Fig. 17b,c ). Altogether, these results indicated that the Tnks-dependent ADP-ribosylation of Axin promotes Axin’s rapid interaction with phospho-LRP6 following Wnt stimulation. Finally, we tested whether the poly(ADP-ribosyl) polymerase (PARP) activity of Tnks promotes the initial activation of Wnt signalling. We generated HA-tagged Tnks transgenes for expression in Drosophila embryos: one transgene encoded wild-type Tnks, whereas the other transgene was identical, except for a methionine to valine substitution (M1064V) in the catalytic PARP domain ( Fig. 8a ). The analogous mutation (M1054V) in the highly conserved PARP domain of human Tnks2 is known to abolish its catalytic activity [58] . Both Tnks transgenes were integrated at the same genomic site, and expressed using the mat-Gal4 driver. As noted above, in Tnks null mutant embryos expressing Axin-V5 , the Wg-dependent expression of engrailed was disrupted ( Fig. 4f ). In contrast, engrailed expression was fully restored in Tnks mutant embryos expressing the wild-type Tnks transgene ( Fig. 8b ), but not the Tnks M1064V transgene ( Fig. 8c ). Together, these findings support the conclusion that the ADP-ribosylation of Axin by Tnks promotes not only the interaction between Axin and phospho-LRP6 following Wg exposure, but also the initial activation of Wg signalling. 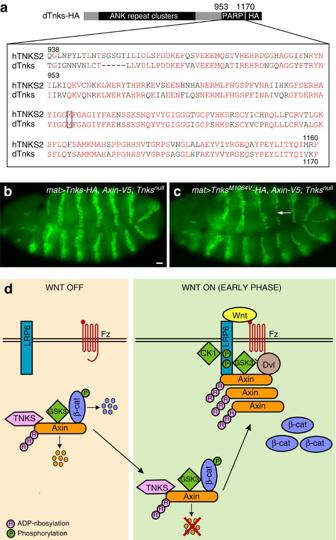Figure 8: Tnks catalytic activity promotes activation of the Wg pathway. (a) Schematic representation of HA-taggedDrosophilaTnks (dTnks-HA). Alignment below shows amino-acid conservation in the catalytic PARP domain of human andDrosophilaTnks. Identical amino acids are in red. Box indicates the substitution indTnksM1064Vthat is predicted to inactivate PARP activity. (b,c) Wg signalling in theTnksnull mutant is rescued by expression of wild-type Tnks, but not catalytically inactive Tnks. Stage 9 embryos stained with En antibody. (b) InTnksnull mutant embryos expressingTnks-HAandAxin-V5driven by themat-Gal4driver, the width of the En stripes is normal (2–3 cells in width). (c) InTnksnull mutant embryos expressingTnksM1064V-HA and Axin-V5driven by themat-Gal4driver, En stripes are aberrantly narrowed (arrow). Scale bar, 25 μm. (d) Model for the dual roles of Tnks in Wnt signalling. Tnks-dependent ADP-ribosylation not only targets Axin for proteolysis independently of Wnt stimulation, but also promotes signalling immediately following Wnt exposure. Wnt stimulation induces the rapid accumulation of ADP-ribosylated Axin. ADP-ribosylation promotes Axin’s interaction with the Wnt co-receptor LRP6, thereby activating the Wnt pathway. Figure 8: Tnks catalytic activity promotes activation of the Wg pathway. ( a ) Schematic representation of HA-tagged Drosophila Tnks ( dTnks-HA ). Alignment below shows amino-acid conservation in the catalytic PARP domain of human and Drosophila Tnks. Identical amino acids are in red. Box indicates the substitution in dTnks M1064V that is predicted to inactivate PARP activity. ( b , c ) Wg signalling in the Tnks null mutant is rescued by expression of wild-type Tnks, but not catalytically inactive Tnks. Stage 9 embryos stained with En antibody. ( b ) In Tnks null mutant embryos expressing Tnks-HA and Axin-V5 driven by the mat-Gal4 driver, the width of the En stripes is normal (2–3 cells in width). ( c ) In Tnks null mutant embryos expressing Tnks M1064V -HA and Axin-V5 driven by the mat-Gal4 driver, En stripes are aberrantly narrowed (arrow). Scale bar, 25 μm. ( d ) Model for the dual roles of Tnks in Wnt signalling. Tnks-dependent ADP-ribosylation not only targets Axin for proteolysis independently of Wnt stimulation, but also promotes signalling immediately following Wnt exposure. Wnt stimulation induces the rapid accumulation of ADP-ribosylated Axin. ADP-ribosylation promotes Axin’s interaction with the Wnt co-receptor LRP6, thereby activating the Wnt pathway. Full size image We demonstrate that Wnt exposure induces biphasic regulation in the level of Axin, and a large increase in the level of ADP-ribosylated Axin immediately after stimulation. ADP-ribosylation enhances the interaction of Axin with phospho-LRP6, and promotes the activation of Wnt signalling. Our findings lead to three major revisions of the current model for the role of Tnks in the activation of the Wnt pathway. First, Tnks serves bifunctional roles under basal conditions and after stimulation, revealing a remarkable economy and coordination of pathway components. Second, our results provide a mechanistic basis for the rapid reprogramming of Axin function in response to Wnt stimulation, and thereby reveal an unanticipated role for Tnks in this process ( Fig. 8d ). These findings suggest that Wnt exposure either rapidly increases the ADP-ribosylation of Axin or inhibits the targeting of ADP-ribosylated Axin for proteasomal degradation, through mechanisms yet to be elucidated. Finally, we demonstrate that pharmacologic inactivation of Tnks diminishes the interaction of Axin with LRP6, revealing a previously unknown mechanism through which small molecule Tnks inhibitors disrupt Wnt signalling, distinct from their known role in stabilizing the destruction complex. In the absence of Wnt stimulation, the concentration-limiting levels of Axin regulate its scaffold function in the destruction complex [15] , [16] . As components of the destruction complex participate in other signalling pathways, the low levels of Axin were proposed to maintain modularity of the Wnt pathway [16] . Our new findings indicate that Axin levels are not only regulated in the absence of Wnt, but also regulated biphasically following Wnt stimulation. This sequential modulation of Axin divides activation of the pathway into an early, fast phase and a delayed long-term phase. During embryogenesis, the earliest expression of Wg triggers the rapid appearance of Axin in segmental stripes, which is a novel hallmark for the initial activation of the pathway. Our findings reveal that Wnt exposure induces a rapid increase in the total level of Axin, and importantly, a preferential increase in the level of the ADP-ribosylated Axin. The early Axin stripes are absent in Tnks null mutant embryos and are also absent when the Tnks binding domain in Axin is deleted. Therefore, we propose that Axin ADP-ribosylation contributes to Axin stabilization and to the rapid response to Wg stimulation. We postulate that the initial increase in levels of ADP-ribosylated Axin jump-starts the response to Wnt stimulation by enhancing the Axin-LRP6 interaction, whereas the subsequent decrease in Axin levels prolongs the duration of signalling by reducing destruction complex assembly. Thus, Wnt stimulation induces rapid increases in the levels of not only cytoplasmic β-catenin, but also ADP-ribosylated Axin. Previous work that coupled mathematical modelling with experimental analysis revealed that several Wnt signalling systems were responsive to the relative change in β-catenin levels, rather than their absolute value [59] . This dependence was proposed to impart robustness and resistance to noise and cellular variation. Our data raise the possibility that a similar principle applies to changes in Axin levels on the Axin-LRP6 interaction, as the marked increase in ADP-ribosylated Axin levels following Wnt stimulation is evolutionarily conserved. Thus, the relative change in levels of ADP-ribosylated Axin may promote signalling following Wnt exposure by facilitating the fold change in β-catenin levels. Our findings have relevance for the context-specific in vivo roles of Tnks in Wnt signalling suggested in previous studies. Tnks inhibition disrupts Wnt signalling in a number of cultured cell lines [28] , but in vivo studies in several model organisms suggested that the requirement for Tnks in promoting Wnt signalling is restricted to specific cell types or developmental stages. In mice, functional redundancy exists between the two Tnks homologues [60] , such that Tnks single mutants are viable and fertile, whereas double mutants display embryonic lethality without overt Wnt-related phenotypes [60] (see Discussion in ref. 61 ). However, a missense mutation in the TBD of Axin2 that is predicted to disrupt ADP-ribosylation resulted in either activating or inhibiting effects on Wnt signalling that were dependent on developmental stage. Tnks inhibitors resulted in the same paradoxical effects, suggesting complex roles in mouse embryonic development [61] . Analogously, treatment of fish with Tnks inhibitors resulted in no observed defects in Wnt-mediated processes during development [28] ; however, the regeneration of injured fins in adults, a process that requires Wnt signalling [62] , was disrupted [28] , [63] . Similarly, the finding that Drosophila Tnks null mutants are viable [49] , [50] , [51] was unexpected, as Tnks is highly evolutionarily conserved, and no other Tnks homologues exist in fly genomes. Nonetheless, our studies reveal that a less than twofold increase in Axin levels uncovers the importance of Tnks in promoting Wg signalling during embryogenesis. Therefore, we postulate that Tnks loss can be compensated during development unless Axin levels are increased, but that the inhibition of Wg signalling resulting from Tnks inactivation cannot be attributed solely to increased Axin levels ( Supplementary Fig. 3 , Figs 4f and 5 ). Furthermore, Drosophila Tnks is essential for Wg target gene activation in the adult intestine, and exclusively within regions of the gradient where Wg is present at relatively low concentration [49] , [64] . Thus, the context-specific roles of Tnks observed in different model organisms may reflect the mechanisms described herein, which reveal that the Wnt-induced association of Axin with LRP6 occurs even in the absence of Axin ADP-ribosylation, but is markedly enhanced in its presence. We postulate that by enhancing this interaction, Tnks-dependent ADP-ribosylation of Axin serves to amplify the initial response to Wnt stimulation, and thus is essential in a subset of in vivo contexts. The recent discovery that Tnks enhances signalling in Wnt-driven cancers has raised the possibility that Tnks inhibitors will offer a promising new therapeutic option [28] , [63] . Indeed, preclinical studies have supported this possibility [30] . Tnks inhibitors were thought previously to disrupt Wnt signalling solely by increasing the basal levels of Axin, and thus by increasing destruction complex activity. However, our findings indicate that the degree to which the basal level of Axin increases following Tnks inactivation is not sufficient to disrupt Wnt signalling in some in vivo contexts. Instead, our results reveal that Tnks inhibition simultaneously disrupts signalling at two critical and functionally distinct steps: by promoting activity of the destruction complex and by diminishing an important step in signalosome assembly: the Wnt-induced interaction between LRP6 and Axin. On the basis of these findings, we propose that the efficacy of Tnks inhibitors results from their combined action at both of these steps, providing a rationale for their use in the treatment of a broad range of Wnt-driven cancers. Therefore, our results suggest that in contrast with the current focus on tumours in which attenuation of the destruction complex aberrantly activates Wnt signalling (such as those lacking APC), the preclinical testing of Tnks inhibitors could be expanded to include cancers that are dependent on pathway activation by Wnt stimulation. These include the colorectal, gastric, ovarian and pancreatic cancers that harbour inactivating mutations in RNF43 (refs 65 , 66 , 67 , 68 , 69 , 70 ), a negative Wnt feedback regulator that promotes degradation of the Wnt co-receptors Frizzled and LRP6 (refs 70 , 71 , 72 ). Drosophila stocks and genetics To generate the pUASTattB Axin-V5 transgene, we isolated a KpnI/HindIII fragment from pAc5.1-Daxin-3xHA (ref. 28 ) and a HindIII/XbaI fragment encoding a triple V5 epitope from pBlue SK-3xV5 (ref. 73 ), and ligated these fragments into pUASTattB (refs 36 , 37 ), at the KpnI and XbaI sites. To generate the pUASTattB-AxinΔTBD-V5 transgene, residues D-12 through K-32 were deleted by PCR-based mutagenesis of pUASTattB-Axin-V5 using the oligonucleotide: 5′-GGTATCTGCTACCCCTTCGGTCATATGTTTCCGGATTCC-3′. The resulting AxinΔTBD-V5 fragment was digested with KpnI and XbaI, and inserted into the pUASTattB vector at the KpnI and XbaI sites. Transgenic flies were generated using phiC31-based integration [36] at the attP33 or attP40 sites on chromosome 2 (ref. 35 ). pUASTattB Axin-GFP was generated using the Gateway LR Clonase system (Invitrogen), with an entry plasmid containing an Axin cDNA amplified by PCR from an ovarian library [74] and the pTWG destination vector containing sequences encoding GFP (Drosophila Genomics Resource Center). Axin-GFP was amplified by PCR using primers that introduced KpnI and XbaI restriction sites at the 5′ and 3′ ends, respectively. Following KpnI and XbaI digestion, the amplified product was cloned into pUASTattB . Transgenic flies were generated using phiC31-based site-specific integration at the attP33 site . Axin-GFP has an 18 amino-acid linker sequence between the carboxy terminus of Axin and the amino terminus of GFP: KPSD/kgradpaflykvvssat/(GFP) (‘/’ represents the junction between Axin and GFP, with additional amino acids shown in lowercase). The pUASTattB-AxinΔTBD-GFP transgene was generated by PCR-based mutagenesis of pUASTattB-Axin-GFP , in which residues D-12 through K-32 were deleted using the oligonucleotide: 5′-GGAATCCGGAAACATATGACCGAAGGGGTAGCAGATACC-3′. The resulting AxinΔTBD-GFP fragment was digested with KpnI and XbaI and inserted into the pUASTattB vector at the KpnI and XbaI sites. To generate the pUASTattB Tnks-HA transgene, a PCR fragment encoding Tnks was amplified from the cDNA LD22548 (Drosophila Genomics Research Center), with the addition of an XhoI restriction site to 5′ end using the primer 5′-ACTCTCGAGATGGCCAACAGCAGCCGAAGT-3′. A fragment encoding a double-HA epitope followed by a KpnI restriction site was added to the 3′ end of the Tnks cDNA using the PCR primer 5′-CATAGTCCGGGACGTCATAGGGATAGCCCGCATAGTCAGGAACATC-3′. The Tnks-HA fragment was digested with XhoI and KpnI, and inserted into the pUASTattB vector at the XhoI and KpnI sites. pUASTattB Tnks M1064V -HA was generated by replacing the methionine at position 1,064 with valine by PCR-based mutagenesis of pUAST-Tnks-2 × HA using the oligonucleotide 5′-ATTGGCGGCGTGTTTGGGGCT-3′, and cloned into the XhoI and KpnI restriction sites of pUASTattB. Transgenic flies were generated using phiC31-based integration at the attP40 site. To obtain embryos expressing Axin-V5 driven by mat-Gal4 : mat-Gal4 females were crossed to UAS-Axin-V5 males. F1 female progeny of the genotype UAS-Axin-V5 / mat-Gal4 were crossed to UAS-Axin-V5 males. To obtain Tnks null mutant embryos expressing Axin-V5 driven by mat-Gal4 : UAS-Axin-V5; Tnks 19 mutant males were crossed to mat-Gal4; Tnks 19 females. F1 female progeny of the genotype UAS-Axin-V5/mat-Gal4; Tnks 19 were crossed to UAS-Axin-V5 ; Tnks 19 males. To obtain Tnks null mutant embryos expressing Tnks-HA and Axin-V5 driven by mat-Gal4 : UAS-Tnks-HA , UAS-Axin-V5 ; Tnks 503 mutant males were crossed to mat-Gal4; Tnks 503 females. F1 female progeny of the genotype UAS-Tnks-HA , UAS-Axin-V5/mat-Gal4 ; Tnks 503 were crossed to UAS-Tnks-HA , UAS-Axin-V5 ; Tnks 503 males. To obtain Tnks null mutant embryos expressing Tnks M1064V -HA and Axin-V5 driven by mat-Gal4: UAS-Tnks M1064V -HA, UAS-Axin-V5; Tnks 503 mutant males were crossed to mat-Gal4; Tnks 503 females. F1 female progeny of the genotype UAS-Tnks M1064V -HA, UAS-Axin-V5/mat-Gal4; Tnks 503 were crossed to UAS-Tnks M1064V -HA, UAS-Axin-V5; Tnks 503 males. Antibodies The primary antibodies used for immunostaining were rabbit anti-V5 (1:1,000, Abcam, ab9116), rabbit anti-GFP (1:200, Invitrogen, A11122), mouse anti-Engrailed (1:100, concentrated 4D9; Developmental Studies Hybridoma Bank, DSHB), mouse anti-Wg (1:200, 4D4 concentrated antibody, DSHB), mouse anti-Arm (1:20, N2 7A1, DSHB) and mouse anti-Neurotactin (1:20, BP106, DSHB). Secondary antibodies were goat or donkey Alexa Fluor 488 or 555 conjugates (1:400, Invitrogen, A21202, A11008, A31572, A31570). The primary antibodies used for immunoblotting were mouse anti-V5 (1:5,000, Invitrogen, 46-1157), guinea pig anti-Axin (1:1,000 (ref. 49 )), mouse anti-Wg (1:100, 4D4, DSHB), rabbit anti-Kinesin Heavy Chain (1:10,000, Cytoskeleton, AKIN01), mouse anti-Arm (1:100, N2 7A1, DSHB), mouse anti-α-Tubulin (1:10,000, DM1A, Sigma, T6199), rabbit anti-α-Tubulin (1:10,000, Sigma, SAB3501071), mouse anti-Flag M2 (1:1000, Sigma, F3165), rabbit anti-GSK3β (1:1,000, Cell Signaling, 9315), mouse anti-β-catenin (1:4,000, BD Biosciences, 610154), rabbit anti-Axin1 (1:1,000, Cell Signaling, #2074), rabbit anti-LRP6 (1:1,000, Cell Signaling, 2560), rabbit anti-c-Myc (1:1,000, Santa Cruz Biotechnology, sc-40), rabbit anti-phospho-LRP6 [Ser1490] (1:1,000, Cell Signaling [8] , 2568), rabbit anti-phospho-LRP6 [Thr1572] (1:1,000, Millipore [44] , 07-2187), and guinea pig anti-Arrow (1:1,000 (ref. 75 )). Secondary antibodies used for immunoblotting were goat anti-rabbit HRP conjugate (1:10,000, Biorad, 170-6515), goat anti-mouse HRP conjugate (1:10,000, Biorad, 170-6516) and goat anti-guinea pig HRP conjugate (1:10,000, Jackson ImmunoResearch). GST-WWE pull downs For GST pull downs, GST-WWE and GST-WWE R164A beads were generated as described previously [52] . Embryos, S2R+ or HEK293T cells were treated as indicated, then washed once with cold 1 × PBS and lysed in lysis buffer (50 mM Tris-HCl [pH 8.0], 100 mM NaCl, 1% NP-40, 10% glycerol, 1.5 mM EDTA [pH 8.0]) or RIPA buffer (50 mM Tris-HCl (pH 8.5), 300 mM NaCl, 1% NP-40, 0.5% sodium deoxycholate and 0.1% SDS) supplemented with 1 μM of the poly(ADP-ribose) glycohydrolase inhibitor ADP-HDP (Enzo Life Sciences), and protease and phosphatase inhibitor cocktail (1:100, Thermo Scientific). Lysates were incubated with GST-WWE or GST-WWE R164A beads overnight at 4 °C. Following incubation, beads were washed four times in wash buffer (50 mM Tris-HCl [pH 8.0], 150 mM NaCl, 1% NP-40, 10% Glycerol, 1.5 mM EDTA [pH 8.0]) supplemented with 1 μM ADP-HPD and protease and phosphatase inhibitor cocktail (1:100). Bound materials were eluted with 2 × sample buffer and resolved by SDS–PAGE, transferred to PVDF or nitrocellulose membranes and blotted with the indicated antibodies. Plasmids Plasmids used for transfection of human cell lines were pCS2+ Flag-mouse Axin1 (ref. 8 ) and pCS2+ Flag-mouse Axin1ΔTBD . To generate the pCS2+ Flag-mouse Axin1ΔTBD plasmid, residues P-26 through E-34 were deleted by PCR-based mutagenesis of pCS2+ Flag-mouse Axin1 using the oligonucleotide: 5′-GATGCCGGAGAACTGGTATCTACTGAT-3′. The resulting Flag-mouse AxinΔTBD fragment was digested with ClaI and BglII, and then inserted into the pCS2+ vector at the ClaI and BglII sites. Plasmids used for transfection of Drosophila cells were pAc5.1-Axin-V5 and pAc5.1-AxinΔTBD-V5 . To generate the pAc5.1-Axin-V5 and pAc5.1-AxinΔTBD-V5 plasmids: fragments encoding Axin-V5 and AxinΔTBD-V5 from pUASTattB-Axin-V5 and pUASTattB-AxinΔTBD-V5 , respectively, were digested using KpnI and XbaI. The resulting fragments were inserted into the pAc5.1 vector (Invitrogen) at the KpnI and XbaI sites. Study design and statistical anaysis In all experiments reported in this study, Student’s t -test and ANOVA test were performed using Prism (GraphPad Software Inc., CA, USA) or the SAS version 9.4 (Statistical Analysis System Institute Inc., NC, USA). Student’s t -test was used to compare two groups for all data sets. ANOVA test was used for comparison of more than two groups. P values and detailed test statistics are provided in the figure legends. No blinding was done and no particular randomization method was used. All experiments were performed at least three times. Additional methods and fly stocks used are described in Supplementary Information . How to cite this article: Yang, E. et al . Wnt pathway activation by ADP-ribosylation. Nat. Commun. 7:11430 doi: 10.1038/ncomms11430 (2016).